Isolation and reversible dimerization of a selenium–selenium three-electron σ-bond Three-electron σ-bonding that was proposed by Linus Pauling in 1931 has been recognized as important in intermediates encountered in many areas. A number of three-electron bonding systems have been spectroscopically investigated in the gas phase, solution and solid matrix. However, X-ray diffraction studies have only been possible on simple noble gas dimer Xe ∴ Xe and cyclic framework-constrained N ∴ N radical cations. Here, we show that a diselena species modified with a naphthalene scaffold can undergo one-electron oxidation using a large and weakly coordinating anion, to afford a room-temperature-stable radical cation containing a Se ∴ Se three-electron σ-bond. When a small anion is used, a reversible dimerization with phase and marked colour changes is observed: radical cation in solution (blue) but diamagnetic dimer in the solid state (brown). These findings suggest that more examples of three-electron σ-bonds may be stabilized and isolated by using naphthalene scaffolds together with large and weakly coordinating anions. Odd-electron species exist as intermediates in many chemical reactions and play an important role in bond formation and cleavage processes [1] , [2] , [3] , [4] , [5] , [6] , [7] . Odd-electron bonding is of both fundamental and practical interest [8] , [9] , [10] , [11] , [12] , [13] . Three-electron σ-bonding was first proposed by Linus Pauling in 1931 (ref. 14 ) and has been recognized as important in major intermediates encountered in many areas such as radical chemistry, biochemistry, organic reactions and radiation studies [15] , [16] , [17] , [18] , [19] , [20] , [21] , [22] . Three-electron σ-bonds are most frequently observed in radical cations ( Fig. 1a ), where they are formed by the interaction of an unpaired electron in a p-orbital of a radical cation with a free p-electron pair from an unoxidized atom, featuring a long weak 2c–3e bond with an antibonding orbital occupied by a single electron and a bond order of 0.5 (hemi-bond). Structure determination and analysis is one of the most useful and direct methods for studies of odd-electron bonds. Although many three-electron σ-bonding systems X ∴ X and X ∴ Y (X, Y=He, N, S, P, halogen and so on) have been investigated in the gas phase, solution and solid matrix, and characterized by various spectroscopic techniques in conjunction with theoretical calculations [23] , [24] , [25] , [26] , [27] , [28] , [29] , [30] , [31] , few of them are room-temperature stable because they are either too reactive or dimerize in the solid state. Only three examples have been isolated and structurally characterized by single-crystal X-ray diffraction ( Fig. 1b ). Gerson et al . [32] and Alder et al . [33] reported cyclic framework-constrained N ∴ N three-electron σ-bonds almost 30 years ago. In 1997, Drews and Seppelt [34] isolated and structurally characterized the Xe 2 + ion containing a Xe ∴ Xe three-electron σ-bond. 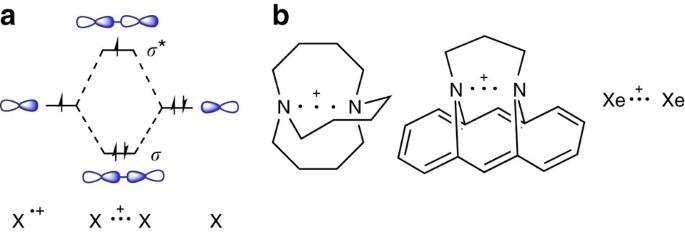Figure 1: Orbital interaction diagram and crystallographically characterized three-electron σ-bonds. (a) Interaction diagram for the formation of a three-electron σ-bond between a radical cation and a neutral atom. (b) Crystallographically characterized three-electron σ-bonds. Figure 1: Orbital interaction diagram and crystallographically characterized three-electron σ-bonds. ( a ) Interaction diagram for the formation of a three-electron σ-bond between a radical cation and a neutral atom. ( b ) Crystallographically characterized three-electron σ-bonds. Full size image We recently have succeeded in stabilization of a number of interesting radical cations [35] , [36] , [37] , [38] , [39] , [40] by using the weakly coordinating anion [Al(OR F ) 4 ] − (OR F =OC(CF 3 ) 3 ) [41] . Inspired by those previous results, we herein report the isolation and structure of a Se ∴ Se three-electron σ-bond, as well as its reversible dimerization. The products were consequently investigated by ultraviolet–visible, electron paramagnetic resonance (EPR), single-crystal X-ray diffraction and superconducting quantum interference device (SQUID) measurements, in conjunction with density functional theory (DFT) calculations. Isolation of radical cation 1 ·+ 1,8-Dichalcogen naphthalene derivatives have been shown to undergo one- and two-electron oxidations by concentrated H 2 SO 4 to form radical cations and dications [42] , [43] , [44] . The unstable radical cations are suggested to contain a Se ∴ Se three-electron σ-bond [42] . Cyclic voltammetry (CV) of 1,8-bis(phenylselenyl)naphthalene (NapSe 2 Ph 2 , 1 ) [45] in CH 2 Cl 2 at room temperature with n -Bu 4 NPF 6 as a supporting electrolyte revealed reversible oxidation peaks at oxidation potentials of +0.94 and +1.15 V ( Supplementary Fig. 1 ). In the light of these CV data, 1 was treated with one equiv NO[Al(OR F ) 4 ] [46] in CH 2 Cl 2 to afford blue radical cation 1 ·+ in a high yield. The resulting cation is thermally stable under nitrogen atmosphere and can be stored for several months at room temperature. Crystals suitable for X-ray crystallographic studies were obtained by cooling a solution of 1 ·+ [Al(OR F ) 4 ] − in CH 2 Cl 2 . Radical cation 1 ·+ is stacked as a dimeric pair ( Supplementary Fig. 2 ) by four Se–C naphthalene contacts (3.55 Å, 2 × ; 3.60 Å, 2 × ) that are close to the sum (3.60 Å) of van der Waals radii of selenium and carbon. In the structure of radical cation 1 ·+ , the naphthalene skeleton is essentially coplanar with two selenium atoms ( Fig. 2 ). This is different from neutral 1 where considerable displacement of the selenium atoms from the naphthyl plane is observed ( Supplementary Fig. 3 ). In 1 ·+ , the phenyl rings overlap in a face-to-face offset arrangement with centroid−centroid distance (3.651(1) Å) within the range for typical π − π stacking (3.3−3.8 Å). Both Se−C Ph bonds are aligning ‘perpendicular’ to the naphthyl plane. The average C–Se bond lengths are shorter while ∠ C–Se–C angles are slightly larger than those in neutral 1 . The Se–Se separation (2.942(1) Å) is shorter than that (3.135(2) Å) in 1 , but much longer than the Se + –Se + single-bond length (2.382(2) Å) in 1,5-diselenoniabicyclo[3.3.0]octane dication [47] . The planarity of the naphthalene-Se–Se backbone, increase of ∠ C–Se–C angle and decrease of Se–Se distance compared with neutral 1 indicate the presence of a weak Se–Se bonding interaction in 1 ·+ . 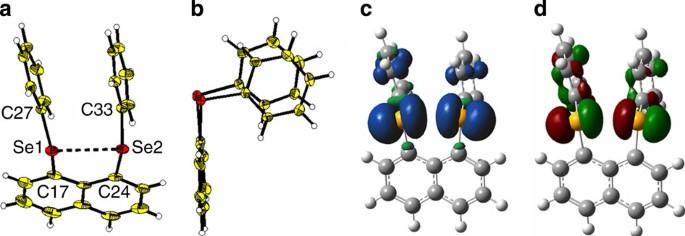Figure 2: Structure, spin-density map and SOMO of 1·+. (a,b) 50% ellipsoid drawings of1·+with different views. Yellow, carbon; red, selenium; white, hydrogen. Selected bond length (Å) and angle (°): Se1–C17 1.915(2), Se1–C27 1.896(2), Se2–C24 1.923(2), Se2–C33 1.909(2), Se1–Se2 2.942(1), C17–Se1–C27 100.65(10), C24–Se2–C33 100.13(10). (c,d) Spin-density map (c) and SOMO (d) for1·+calculated at the UPBE0/SVP level. Figure 2: Structure, spin-density map and SOMO of 1 ·+ . ( a , b ) 50% ellipsoid drawings of 1 ·+ with different views. Yellow, carbon; red, selenium; white, hydrogen. Selected bond length (Å) and angle (°): Se1–C17 1.915(2), Se1–C27 1.896(2), Se2–C24 1.923(2), Se2–C33 1.909(2), Se1–Se2 2.942(1), C17–Se1–C27 100.65(10), C24–Se2–C33 100.13(10). ( c , d ) Spin-density map ( c ) and SOMO ( d ) for 1 ·+ calculated at the UPBE0/SVP level. Full size image To rationalize the experimental results and get further insights into their electronic structures, we carried out DFT calculations for species 1 and 1 ·+ , along with dication 1 2+ . The calculated energy Δ E for the reaction 2 1 ·+ → 1 + 1 2+ in the solution of CH 2 Cl 2 is +24.1 kcal mol −1 , which indicates it is unlikely for the radical cation ( 1 ·+ ) to disproportionate to neutral 1 and dication 1 2+ . X-ray crystal structures of 1 and 1 ·+ were well reproduced by DFT calculations ( Table 1 ; Supplementary Fig. 4 ). Consistent with the experimental data, one-electron oxidation of 1 causes a significant decrease of the Se–Se separation by ~0.2 Å, which combined with dominant spin-density distribution ( Fig. 2c ; Supplementary Table 2 ) on Se atoms (0.427, 0.421) becomes strong evidence for the formation of a 2c–3e hemi-bond between Se atoms. The calculated Mayer bond order (0.360) for Se−Se further supports the hemi-bond formation. As shown in Fig. 2d , both selenium atoms are main contributors to the singly occupied molecular orbital (SOMO), with Se−Se antibonding character. To check whether the naphthalene scaffold affects the Se−Se bonding, model compounds Me 2 SeSeMe 2 ·+ and Ph 2 SeSePh 2 ·+ were also calculated, which afforded linear Se−Se antibonding orbitals with trans configurations ( Supplementary Fig. 5 ). The slight bending of SOMO of 1 ·+ is due to the constraints imposed by the naphthalene scaffold. Table 1 Structural parameters of 1 and 1 ·+ . Full size table The radical and hemi-bond identification was completed by EPR, nuclear magnetic resonance (NMR), SQUID and ultraviolet–visible measurements. The solution EPR spectrum ( Fig. 3a ) of 1 ·+ [Al(OR F ) 4 ] − at 298 K shows 77 Se (spin I=1/2; natural abundance=7.6) satellite peaks, which is attributed to Nap 77 SePhSePh species. The signal for the Nap 77 SePh 77 SePh isotopomer is too weak to observe because of its low concentration. The ratio of main (even-numbered Se isotopes) to satellite ( 77 Se) spectrum intensities is in agreement with the expected value (12.2) and the A iso (95G) is comparable to that for Me 2 SeSeMe 2 ·+ (108G) observed in the γ -irradiated sample [48] . The EPR spectrum of crystalline 1 ·+ [Al(OR F ) 4 ] − shows an anisotropic spectrum with g x =2.0011, g y =2.0255 and g z =2.0441 ( Supplementary Fig. 6 ). The g iso value (2.0236) is close to that of (Me 2 SeSeMe 2 ) ·+ ( g iso =2.0344) [48] but is significantly smaller than those (2.0639–2.0644) of the diaryl diselenide radical cations (ArSeSeAr) ·+ stabilized in pentasil zeolite (Na-ZSM-5) [49] , where a two-center three-electron π–bond is suggested ( Supplementary Fig. 7 ). The paramagnetic property of radical salt 1 ·+ [Al(OR F ) 4 ] − was further confirmed by SQUID measurement ( Supplementary Fig. 8 ) and broad 1 H NMR peaks ( Supplementary Fig. 9 ). The ultraviolet–visible spectrum with broad absorption peaks ( Fig. 3b ) is typical of a three-electron σ-bond and the absorptions are in the range of 370–680 nm for the reported absorptions of S ∴ S and Se ∴ Se bonds in the solution [50] . Judging from the time-dependent DFT calculations of 1 ·+ opt ( Supplementary Fig. 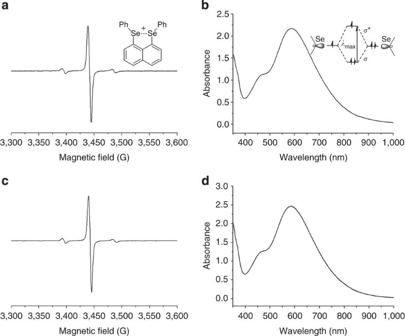Figure 3: Absorption and EPR spectra for 1·+. (a,c) EPR spectra for1·+[Al(ORF)4]−(a) and1·+SbF6−(c) in CH2Cl2(1 × 10−4M, 298 K). (b,d) Absorption spectra for1·+[Al(ORF)4]−(b) and1·+SbF6−(d) in CH2Cl2(1 × 10−4M, 298 K). 10 ; Supplementary Table 3 ), absorptions around 580 ( ε 21750) and 465 nm ( ε 11080) are assigned to overlapped transitions of HOMO(β)→LUMO(β) (I) and HOMO-1(β)→LUMO(β) (II) (580 nm: I 84%, II 12%; 465 nm: I 13%, II 83%). Figure 3: Absorption and EPR spectra for 1 ·+ . ( a , c ) EPR spectra for 1 ·+ [Al(OR F ) 4 ] − ( a ) and 1 ·+ SbF 6 − ( c ) in CH 2 Cl 2 (1 × 10 −4 M, 298 K). ( b , d ) Absorption spectra for 1 ·+ [Al(OR F ) 4 ] − ( b ) and 1 ·+ SbF 6 − ( d ) in CH 2 Cl 2 (1 × 10 −4 M, 298 K). Full size image Dimerization of radical cation 1 ·+ Further experimental work shows that the formation of Se ∴ Se bonding is anion dependent. The reaction of 1 with 1 equiv NOSbF 6 resulted in a blue solution of 1 ·+ SbF 6 − . The ultraviolet–visible absorption, EPR spectra ( Fig. 3c,d ) and broadness of 1 H NMR peak ( Supplementary Fig. 11 ) of the reaction solution are similar to those of 1 ·+ [Al(OR F ) 4 ] − . Compared with the sharp 19 F peak ( δ −75.22 p.p.m.) [51] in the NMR spectrum of 1 ·+ [Al(OR F ) 4 ] − , a very broad 19 F NMR peak is observed in that of 1 ·+ SbF 6 − , suggesting some degree of interaction between ion pairs in the solution of 1 ·+ SbF 6 − ( Supplementary Figs 12 and 13 ). Concentrating and cooling the blue solution of 1 ·+ SbF 6 − afforded reddish brown crystals, which were identified as a dimeric complex [ 1–1 ] 2+ (SbF 6 − ) 2 by X-ray crystallographic analysis. Redissolving [ 1–1 ] 2+ (SbF 6 − ) 2 in CH 2 Cl 2 immediately gave a blue solution with an identical absorption spectrum to 1 ·+ SbF 6 − . The crystallization and dissolution accompanied with intense colour change demonstrate a reversible process between radical cation 1 ·+ and dimer [ 1–1 ] 2+ , as shown in Fig. 4a . The solid [ 1–1 ] 2+ (SbF 6 − ) 2 exhibits an EPR spectrum ( Supplementary Fig. 14 ), which is similar to that observed for 1 ·+ [Al(OR F ) 4 ] − , but a magnetic susceptibility measurement indicates that the brown solid is diamagnetic ( Supplementary Fig. 15 ). The EPR signal of the solid is probably due to trace amounts of radical cation salt 1 ·+ SbF 6 − trapped in the solid. A similar reversible process with colour change from yellow to red was observed during the oxidation of 1,5-dithiacyclooctane, but has not been identified [52] . 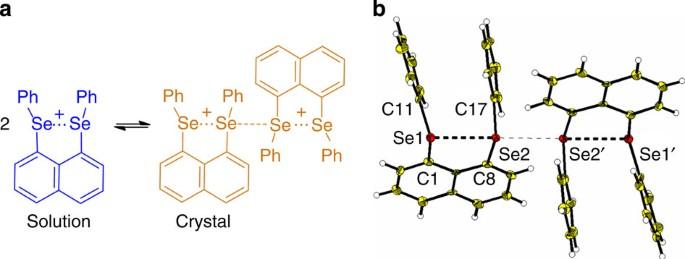Figure 4: Reversible dissociation and crystal structure of [1–1]2+. (a) Reversible dissociation of[1–1]2+. (b) Crystal structure of[1–1]2+(in[1–1]2+(SbF6−)2) with 50% ellipsoid drawing. Yellow, carbon; red, selenium; white, hydrogen. Selected bond length (Å) and angle (°): Se1–C1 1.916(7), Se1–C11 1.912(8), Se2–C8 1.939(7), Se2–C17 1.931(8), Se1–Se2 2.8815(9), Se2–Se2' 2.9543(13), C1–Se1–C11 101.1(3), C8–Se2–C17 100.2(3), Se1–Se2–Se2' 174.79(4), Se1–Se2–Se2'–Se1' −180.0. Figure 4: Reversible dissociation and crystal structure of [1–1] 2+ . ( a ) Reversible dissociation of [1–1] 2+ . ( b ) Crystal structure of [1–1] 2+ (in [1–1] 2+ (SbF 6 − ) 2 ) with 50% ellipsoid drawing. Yellow, carbon; red, selenium; white, hydrogen. Selected bond length (Å) and angle (°): Se1–C1 1.916(7), Se1–C11 1.912(8), Se2–C8 1.939(7), Se2–C17 1.931(8), Se1–Se2 2.8815(9), Se2–Se2' 2.9543(13), C1–Se1–C11 101.1(3), C8–Se2–C17 100.2(3), Se1–Se2–Se2' 174.79(4), Se1–Se2–Se2'–Se1' −180.0. Full size image Single-crystal X-ray diffraction showed that [ 1–1 ] 2+ is composed of two asymmetric subunits symmetrically coupled through a selenium–selenium interaction, giving rise to a linear Se–Se–Se–Se arrangement ( Fig. 4b ). Compared with the structure of radical cation 1 ·+ , the Se1–C bond distances (Se1–C1, Se1–C11) basically keep unchanged, while the Se2–C bonds (Se2–C17, Se2–C8) are lengthened and the intramolecular Se–Se distance (Se1–Se2) of 2.8815(9) becomes shorter. The Se–Se distance (Se2–Se2′ 2.9543 (13) Å) connecting two subunits is quite long. These Se–Se contacts in [ 1–1 ] 2+ are comparable to those (2.715(4)–2.929(2) Å) in donor–acceptor complex cations of selone derivatives with TCNQ reported by Bigoli et al . [53] , Devillanova et al . [54] , in which the nearly linear arrangement of Se–Se–Se is viewed as a three-center two-electron bond. The unusual dimeric structure of [ 1–1 ] 2+ resembles the dimer of unstable tellurium-centered (TePiPr 2 NiPr 2 PTe) · radical [55] . It is also worth noting that dialkyl dichalcogen radical cation (MeSe) 2 ·+ , containing a two-center three-electron Se–Se π-bond, dimerizes as a rectangular species (MeSe) 4 2+ by a π*–π* interaction with long Se–Se bonds (2.974(1) Å) [56] that are comparable to those of [ 1–1 ] 2+ . However, in these cases reversibility was not observed [53] , [54] , [55] , [56] . The crystal structure of the dimer [ 1–1 ] 2+ has been reproduced as a closed-shell singlet by theoretical calculations. Of particular note, the calculated Se2–Se2′ bond lengths (2.9236 Å) is comparable to that (2.9543(13) Å) in the X-ray structure of [ 1–1 ] 2+ . The HOMO clearly shows a σ*–σ* interaction between two radical cation SOMOs ( Fig. 5a ). Notably Se2–Se2′ bond length of [ 1–1 ] 2+ is much longer than that (2.6471(6) Å) of the dicationic dimer by irreversible coupling of hypothetical 1,5-selenathiamesocycle radical cation [57] . The long and weak intermolecular Se–Se bond in [1–1] 2+ (SbF 6 − ) 2 thus accounts for the reversibility of dimerization, and is due to the multicentered nature of the radical SOMO. However, the magnitude of the electronic coupling between the radical cation moieties in the solid state is sufficient to lead to bulk diamagnetism of [ 1–1 ] 2+ as proved by SQUID measurements. In terms of the valence bond theory, the Se–Se–Se–Se fragment in [ 1 – 1 ] 2+ may be viewed as a 4c–6e bonding stabilized by some resonance structures ( Fig. 5b ) [58] . 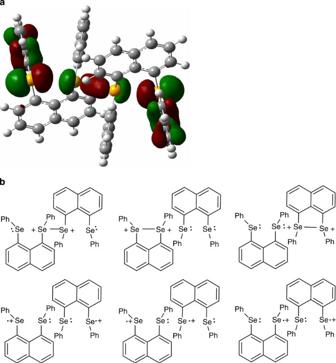Figure 5: Frontier molecular orbital and resonance structures of [1–1]2+. (a) HOMO of[1–1]2+showing a σ*–σ* interaction between two radical cation SOMOs. (b) Resonance structures. Figure 5: Frontier molecular orbital and resonance structures of [1–1] 2+ . ( a ) HOMO of [1–1] 2+ showing a σ*–σ* interaction between two radical cation SOMOs. ( b ) Resonance structures. Full size image We here have shown that the diselena species ( 1 ) modified with a naphthalene scaffold can undergo one-electron oxidation using a large and weakly coordinating anion [Al(OR F ) 4 ] − , to afford a room-temperature-stable radical cation ( 1 ·+ ) containing a Se ∴ Se three-electron σ-bond. When a smaller anion SbF 6 − is used, a reversible dimerization with phase and marked colour changes is observed: radical cation ( 1 ·+ ) in blue solution but brown diamagnetic dimer ([ 1 – 1 ] 2+ ) in the solid state. The energy Δ E calculated at the (U)PBE0/SVP level for the dimerization 2 1 ·+ →[ 1–1 ] 2+ is +37.2 and +3.82 kcal mol −1 in the gas phase and CH 2 Cl 2 solution, respectively, indicating it is thermodynamically unfavourable for 1 ·+ to dimerize in the gas phase or in solution. This is due to the strong electrostatic repulsion of the two adjacent positive charges in [ 1–1 ] 2+ , which is relieved upon dissociation. The unstable dimeric species [ 1–1 ] 2+ in the gas phase is lattice stabilized by the formation of the salt [ 1–1 ] 2+ (SbF 6 − ) 2 in the solid state, because the lattice energy for [ 1–1 ] 2+ (SbF 6 − ) 2 is about three times that of 1 ·+ SbF 6 − assuming ionic radii are similar, as shown by the Kapustiniskii equation ( Fig. 6a ) [41] , [59] , [60] , [61] , where z x and z y are the charge of the ions, r x and r y the ionic radii and ν is the number of ions per formula unit (for example, two for X + Y − and three for X 2+ (Y − ) 2 ). As shown in the Born–Fajans–Haber cycle ( Fig. 6b ), replacement of the anion SbF 6 − (0.121 nm 3 ) by the larger anion [Al(OR F ) 4 ] − (0.736 nm 3 ) leads to a great reduction (less negative) in the lattice energy difference {Δ latt U ([ 1–1 ] 2+ (A − ) 2 )−Δ latt U (2 1 ·+ A − )}, which would make Δ E (s) more positive and thus favours the formation of singly charged 1 ·+ over the doubly charged [ 1–1 ] 2+ . Our findings suggest that more examples of three-electron σ-bonds may be stabilized by using naphthalene scaffolds together with large and weakly coordinating anions. Isolation of other examples of those elusive and intriguing three-electron σ-bonds X ∴ X and X ∴ Y (X, Y=S, Te, P, As, halogen and so on) is under way. 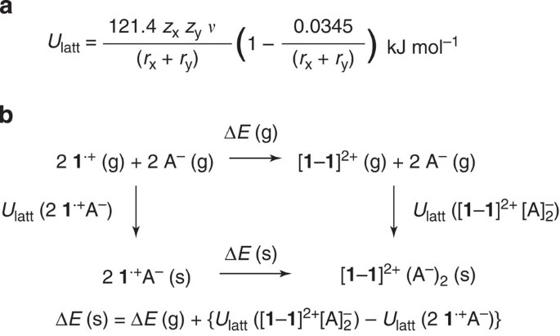Figure 6: Lattice energy estimation and the energetics of the radical dimerization. (a) Kapustiniskii equation for lattice energy estimation. (b) Born–Fajans–Haber cycle rationalizing the formation of the dimer[1–1]2+(A−)2. Figure 6: Lattice energy estimation and the energetics of the radical dimerization. ( a ) Kapustiniskii equation for lattice energy estimation. ( b ) Born–Fajans–Haber cycle rationalizing the formation of the dimer [1–1] 2+ (A − ) 2 . Full size image General All experiments were carried out under a nitrogen atmosphere by using standard Schlenk techniques and a glovebox. Solvents were dried before use. NOSbF 6 (Alfa Aesar) was purchased and used upon arrival. 1,8-bis(phenylselanyl) naphthalene ( 1 ) [45] and NO[Al(OR F ) 4 ] [46] were synthesized according to the literature methods. CV was performed on an IM6ex electrochemical workstation, with platinum as the working and counter electrodes, Ag/Ag + as the reference electrode and 0.1 M n -Bu 4 NPF 6 as the supporting electrolyte. EPR spectra were obtained using the Bruker EMX-10/12 variable-temperature apparatus. ultraviolet–visible spectra were recorded on the Lambda 750 spectrometer. Element analyses were performed at Shanghai Institute of Organic Chemistry, the Chinese Academy of Sciences. Magnetic measurements were performed using a Quantum Design MPMS XL-7 SQUID magnetometer at a temperature ranging from 5 to 350 K. The 1 H NMR spectra were performed using a Bruker DRX-500 spectrometer in p.p.m. downfield from Me 4 Si. 19 F NMR spectra were performed at ambient temperature on the Bruker DRX-400 spectrometer using CFCl 3 as an external reference. X-ray crystal structures were obtained by using a Bruker APEX DUO CCD detector. Crystal data and structure refinement for 1 ·+ [Al(OR F ) 4 ] − and [ 1–1 ] 2+ (SbF 6 − ) 2 are listed in Supplementary Table 1 . Preparation of 1 ·+ [Al(OR F ) 4 ] − Under anaerobic and anhydrous conditions, a mixture of 1 (0.088 g, 0.2 mmol) and NO[Al(OR F ) 4 ](0.199 g, 0.2 mmol) in CH 2 Cl 2 (≈50 ml) was stirred at room temperature for 1 day. The resulting blue solution was then concentrated and stored at around −20 °C for 24 h to afford X-ray-quality crystals of the radical cation salt 1 ·+ [Al(OR F ) 4 ] − . Isolated yield: 0.124 g, 44% (crystals); mp 135–137 °C; ultraviolet–visible (CH 2 Cl 2 ): λ max 465 ( ε 11080, shoulder), 580 ( ε 21750) nm; analysis (calcd., found for C 38 H 16 AlF 36 O 4 Se 2 ) C (32.48, 32.82), H (1.15, 1.26). Preparation of 1 ·+ SbF 6 − and [ 1–1 ] 2+ (SbF 6 − ) 2 Under anaerobic and anhydrous conditions, a mixture of 1 (0.132 g, 0.3 mmol) and NOSbF 6 (0.080 g, 0.3 mmol) in CH 2 Cl 2 (≈50 ml) was stirred at room temperature for 1 day. The resulting blue solution of 1 ·+ SbF 6 − was then concentrated and stored at around −20 °C for 24 h to afford X-ray-quality crystals of salt [1–1] 2+ (SbF 6 − ) 2 . Isolated yield: 0.103 g, 45% (crystals); mp 153–155 °C; ultraviolet–visible (CH 2 Cl 2 ): λ max 460 ( ε 12190, shoulder), 588 ( ε 24320) nm; analysis (calcd., found for C 44 H 32 F 12 Sb 2 Se 4 · CH 2 Cl 2 ): C (37.72, 38.15), H (2.39, 2.57). Quantum chemical calculations Calculations were performed with the Gaussian 09 program suite ( Supplementary Note 1 ; Supplementary Reference 2 ). Geometries were optimized and checked as energy minima by frequency calculations at the (U)PBE0/SVP level of theory. The ultraviolet–visible absorption spectrum was calculated on the optimized geometry using the time-dependent DFT method at the UM06-2X/6-31+G(d) level. To consider solvent (CH 2 Cl 2 ) effects, a polarized continuum model was adopted in the calculation of the single-point energies involved in the the disproportionation and dimerization, and ultraviolet–visible absorption spectrum. Mayer bond order was calculated at the UPBE0/SVP level with the Multiwfn program [62] . How to cite this article: Zhang, S. et al . Isolation and reversible dimerization of a selenium–selenium three-electron σ-bond. Nat. Commun. 5:4127 doi: 10.1038/ncomms5127 (2014).